Shared heritability and functional enrichment across six solid cancers Quantifying the genetic correlation between cancers can provide important insights into the mechanisms driving cancer etiology. Using genome-wide association study summary statistics across six cancer types based on a total of 296,215 cases and 301,319 controls of European ancestry, here we estimate the pair-wise genetic correlations between breast, colorectal, head/neck, lung, ovary and prostate cancer, and between cancers and 38 other diseases. We observed statistically significant genetic correlations between lung and head/neck cancer ( r g = 0.57, p = 4.6 × 10 −8 ), breast and ovarian cancer ( r g = 0.24, p = 7 × 10 −5 ), breast and lung cancer ( r g = 0.18, p =1.5 × 10 −6 ) and breast and colorectal cancer ( r g = 0.15, p = 1.1 × 10 −4 ). We also found that multiple cancers are genetically correlated with non-cancer traits including smoking, psychiatric diseases and metabolic characteristics. Functional enrichment analysis revealed a significant excess contribution of conserved and regulatory regions to cancer heritability. Our comprehensive analysis of cross-cancer heritability suggests that solid tumors arising across tissues share in part a common germline genetic basis. Inherited genetic variation plays an important role in cancer etiology. Large twin studies have demonstrated an excess familial risk for cancer sites including, but not limited to, breast, colorectal, head/neck, lung, ovary, and prostate with heritability estimates ranging between 9% (head/neck) to 57% (prostate) [1] , [2] , [3] . Data from nation-wide and multi-generation registries further show that elevated cancer risks go beyond nuclear families and isolated types, as family history of a specific cancer can increase risk for other cancers [4] , [5] , [6] . Additional evidence for a shared genetic component have been demonstrated by cross-cancer genome-wide association study (GWAS) meta-analyses, which set out to identify genetic variants associated with more than one cancer type. Fehringer et al. studied breast, colorectal, lung, ovarian, and prostate cancer, and identified a novel locus at 1q22 associated with both breast and lung cancer [7] . Kar et al. focused on three hormone-related cancers (breast, ovarian, and prostate), and identified seven novel susceptibility loci shared by at least two cancers [8] . Previous attempts to estimate the genetic correlation across cancers using GWAS data [9] , [10] , [11] , [12] have mostly relied on restricted maximum likelihood (REML) implemented in GCTA (genome-wide complex trait analysis) [13] and individual-level genotype data. However, these studies have had limited sample sizes, yielding inconclusive results. Sampson et al. quantified genetic correlations across 13 cancers in European ancestry populations and identified four cancer pairs with nominally significant genetic correlations (bladder–lung, testis–kidney, lymphoma–osteosarcoma, and lymphoma–leukemia) [9] . They did not observe any significant genetic correlations across common solid tumors including cancers of the breast, lung and prostate [9] . REML becomes computationally challenging for large sample sizes and is sensitive to technical artifacts. LD score regression (LDSC) [14] , [15] overcomes these issues by leveraging the relationship between association statistics and LD patterns across the genome. We recently used cross-trait LDSC to quantify genetic correlations across six cancers based on a subset of the data included here and found moderate correlations between colorectal and pancreatic cancer, as well as between lung and colorectal cancer [16] . However, the average sample size was only 11,210 cases and 13,961 controls per cancer, resulting in imprecise estimates with wide confidence intervals. In addition to the development of novel analytical methods tailored to genomic data, several high-quality functional annotations have recently been released into the public domain through large-scale efforts. For example, the ENCODE consortium has built a comprehensive and informative parts list of functional elements in the human genome ( http://www.nature.com/encode/#/threads ), which allows for the analysis of components of SNP-heritability to unravel the functional architecture of complex traits. Here, we use summary statistics from the largest-to-date European ancestry GWAS of breast, colorectal, head/neck, lung, ovary, and prostate cancer with an average sample size of 49,369 cases and 50,219 controls per cancer, to quantify genetic correlations between cancers and their subtypes. We also use GWAS summary statistics for 38 non-cancer traits (average N = 113,808 per trait), to quantify the genetic correlations between the six cancers and other diseases. Furthermore, we assessed the proportion of cancer heritability attributable to specific functional categories, with the goal of identifying functional elements that are enriched for SNP-heritability. Our comprehensive analysis identifies statistically significant genetic correlations between lung and head/neck cancer, breast and ovarian cancer, breast and lung cancer, and breast and colorectal cancer. We also find multiple cancers to be genetically correlated with non-cancer traits including smoking, psychiatric diseases, and metabolic traits. Functional enrichment analysis reveals a significant contribution of conserved and regulatory regions to cancer heritability. Our results suggest that solid tumors arising across tissues share in part a common germline genetic basis. Heritability estimates across cancers We first estimated cancer-specific heritability causally explained by common SNPs ( \(h_g^2\) ) using LDSC (note that this quantity is slightly different from the \(h_g^2\) as defined in Yang et al. [17] which estimates the heritability due to genotyped and imputed SNPs) (see Methods). 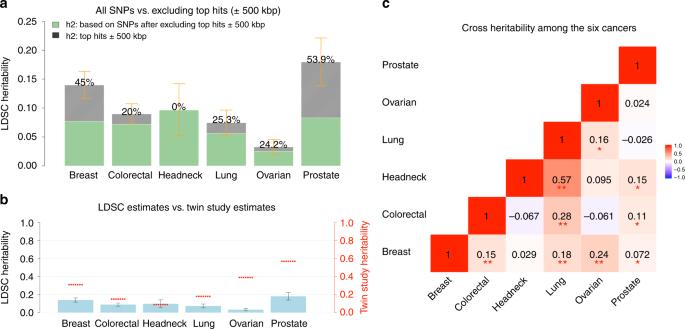Fig. 1 Estimates of SNP-heritability (\(h_g^2\)) and cross-cancer heritability (rg) for the six cancer types. SNP-heritability and cross-cancer heritability are calculated based on HapMap3 SNPs using LD score regression (LDSC).aThe solid bar represents overall SNP\(h_g^2\)on the liability scale, calculated based on all HapMap3 SNPs. The dark green bar represents\(h_g^2\)calculated based on non-significant SNPs—the remaining SNPs after excluding genome-wide significant hits (p< 5 × 10−8) ± 500 kb. The black bar with density texture indicates proportion of\(h_g^2\)(as reflected by the percentages displayed on top of each bar) that could be explained by top hits ±500 kb surrounded areas. The orange error bars represent 95% confidence intervals.bThe solid blue bar represents overall SNP\(h_g^2\)in liability scale (no SNP exclusion), with black error bars indicating 95% confidence intervals. The red short lines correspond to classical estimates ofh2measured in a twin study of Scandinavian countries (Mucci et al.2).cGenetic correlations between cancers. Estimates withstood Bonferroni corrections (p< 0.05/15) are marked with double asterisk (**), and nominal significant results (p< 0.05) are marked with single asterisk (*) Estimates of \(h_g^2\) on the liability scale ranged from 0.03 (ovarian) to 0.25 (prostate) (Supplementary Table 1 ). After removing genome-wide significant ( p < 5 × 10 −8 ) loci, defined as all SNPs within 500 kb of the most significant SNP in a given region (Supplementary Data 1 ), we observed an ~50% decrease in SNP-heritability for prostate and breast cancer, and ~20% decrease for lung, ovarian, and colorectal cancer, despite the fact that we were only excluding 1% (colorectal cancer) to 5% (breast cancer) of the genome. In contrast, the SNP-heritability for head/neck cancer was not affected by removing genome-wide significant loci (Fig. 1a ). For most of the cancers, the GWAS significant loci for that particular cancer explained most of the heritability. For some cancers, however, significant GWAS loci of other cancers also explained a non-trivial part of its heritability. 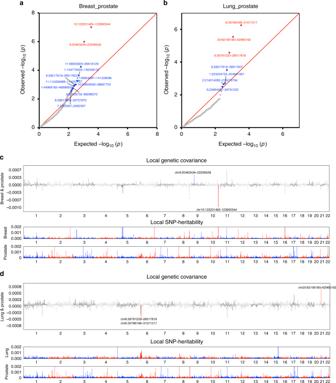Fig. 2 Local genetic correlation between breast, lung and prostate cancer. The region-specificp-values for the local genetic covariance for breast and prostate cancer are shown ina, and for lung and prostate cancer inb. Each dot presents a specific genomic region. In the QQ plots, red color indicates significance after multiple corrections (p< 0.05/1703 regions compared), and blue color indicates nominal significance (p< 0.05/15 pairs of cancers compared). Manhattan-style plots showing the estimates of local genetic covariance for breast and prostate cancer (c), and for lung and prostate cancer (d). Although breast and prostate cancer only show modest genome-wide genetic correlation, two loci exhibit significant local genetic covariance. Similarly, albeit the negligible overall genetic correlation for lung and prostate cancer, three loci present significant local genetic covariance. In the Manhattan plots, red color indicates even number chromosomes and blue color indicates odd number chromosomes For example, the significant breast cancer GWAS loci explained 10%, 15%, and 22% heritability of colorectal, ovarian and prostate cancer, respectively; the significant colorectal cancer GWAS loci explained 11% heritability of prostate cancer; the significant lung cancer GWAS loci explained 10% heritability of head/neck cancer; and the significant prostate cancer GWAS loci explained 11 and 15% heritability of breast and ovarian cancer, respectively (Supplementary Table 2 ). Comparing the liability-scale SNP-heritability to corresponding estimates from twin studies suggests that common SNPs can almost entirely explain the classical heritability of head/neck cancer, whereas for other cancers, only 30–40% of heritability can be explained (Fig. 1b ). Fig. 1 Estimates of SNP-heritability ( \(h_g^2\) ) and cross-cancer heritability ( r g ) for the six cancer types. SNP-heritability and cross-cancer heritability are calculated based on HapMap3 SNPs using LD score regression (LDSC). a The solid bar represents overall SNP \(h_g^2\) on the liability scale, calculated based on all HapMap3 SNPs. The dark green bar represents \(h_g^2\) calculated based on non-significant SNPs—the remaining SNPs after excluding genome-wide significant hits ( p < 5 × 10 −8 ) ± 500 kb. The black bar with density texture indicates proportion of \(h_g^2\) (as reflected by the percentages displayed on top of each bar) that could be explained by top hits ±500 kb surrounded areas. The orange error bars represent 95% confidence intervals. b The solid blue bar represents overall SNP \(h_g^2\) in liability scale (no SNP exclusion), with black error bars indicating 95% confidence intervals. The red short lines correspond to classical estimates of h 2 measured in a twin study of Scandinavian countries (Mucci et al. [2] ). c Genetic correlations between cancers. Estimates withstood Bonferroni corrections ( p < 0.05/15) are marked with double asterisk (**), and nominal significant results ( p < 0.05) are marked with single asterisk (*) Full size image Genetic correlations between cancers We then estimated the genetic correlation between cancers using cross-trait LDSC (see Methods). After adjusting for the number of tests ( p < 0.05/15 = 0.003), we found multiple significant genetic correlations Fig. 1c and Supplementary Table 1 ), with the strongest result observed for lung and head/neck cancer ( r g = 0.57, se = 0.10). In addition, colorectal and lung cancer ( r g = 0.28, se = 0.06), breast and ovarian cancer ( r g = 0.24, se=0.06), breast and lung cancer ( r g = 0.18, se = 0.04), and breast and colorectal cancer ( r g = 0.15, se = 0.04) showed statistically significant genetic correlations. We also observed nominally significant genetic correlations ( p < 0.05) between lung and ovarian cancer ( r g = 0.16, se = 0.08), prostate cancer and head/neck ( r g = 0.15, se = 0.08), colorectal ( r g = 0.11, se = 0.05), and breast cancer ( r g = 0.07, se = 0.03) (Fig. 1c ). Some cancer pairs showed minimal correlations with estimates close to 0 (ovarian and prostate: r g = 0.02, se = 0.07; lung and prostate: r g = −0.03, se = 0.04; breast and head/neck: r g = 0.03, se = 0.06). We further calculated the cross-cancer genetic correlation based on data after excluding the GWAS significant regions of each cancer. The estimates were mostly consistent with the results calculated based on all SNPs. We conducted subtype-specific analysis for breast, lung, ovarian, and prostate cancer (Supplementary Table 1 ). Estrogen receptor positive (ER+) and negative (ER−) breast cancer showed a genetic correlation of 0.60 (se = 0.03), indicating that the genetic contributions to these two subtypes are in part distinct. The genetic correlation between the two common lung cancer subtypes adenocarcinoma and squamous cell carcinoma was similarly 0.58 (se = 0.10). Further, we observed a significantly larger genetic correlation of lung cancer with ER− ( r g = 0.29, se = 0.06) than with ER + breast cancer ( r g = 0.13, se = 0.04) ( p difference = 0.002). This also held true for lung squamous cell carcinoma, which showed statistically stronger genetic correlation with ER− ( r g = 0.33, se = 0.08) than with ER + breast cancer ( r g = 0.11, se = 0.05) ( p difference = 0.0019). We observed no other statistically significant differential genetic correlations across subtypes (all p difference > 0.1). We then estimated local genetic correlations between cancers using ρ-HESS, dividing the genome into 1703 regions (see Methods) (Fig. 2 and Supplementary Fig. 1 ). We found that although the genome-wide genetic correlation between breast and prostate cancer was modest ( r g = 0.07), chr10:123M (10q26.13, p = 1.0 × 10 −7 ) and chr9:20–22 M (9p21, p = 1.0 × 10 −6 ), two previously known pleiotropic regions [18] , showed significant genetic correlations ( r g = −0.00098 and r g = 0.00046). Similarly, although the genome-wide genetic correlation between lung and prostate cancer was negligible ( r g = −0.03), two previously identified pleiotropic regions (chr6:30–31 M or 6p21.33, p = 5.7 × 10 −7 and chr20:62M or 20q13.33, p = 2.8 × 10 −6 ) exhibited significant local genetic correlations ( r g = −0.00060 and r g = 0.00067). Overall, local genetic correlation analysis reinforced shared effects for 44% (31/71) of previously reported pleiotropic cancer regions (Supplementary Data 2 ). It also identified novel pleiotropic signals. For example, the breast and prostate cancer pleiotropic region at 2q33.1 showed significant local genetic correlation between breast and ovarian cancer ( p = 2.3 × 10 −6 ). Additionally, 6p21.32, a region indicated for head/neck and prostate cancer, showed highly significant local genetic correlation for head/neck and lung cancer ( p = 8.6 × 10 −8 ). Fig. 2 Local genetic correlation between breast, lung and prostate cancer. The region-specific p -values for the local genetic covariance for breast and prostate cancer are shown in a , and for lung and prostate cancer in b . Each dot presents a specific genomic region. In the QQ plots, red color indicates significance after multiple corrections ( p < 0.05/1703 regions compared), and blue color indicates nominal significance ( p < 0.05/15 pairs of cancers compared). Manhattan-style plots showing the estimates of local genetic covariance for breast and prostate cancer ( c ), and for lung and prostate cancer ( d ). Although breast and prostate cancer only show modest genome-wide genetic correlation, two loci exhibit significant local genetic covariance. Similarly, albeit the negligible overall genetic correlation for lung and prostate cancer, three loci present significant local genetic covariance. In the Manhattan plots, red color indicates even number chromosomes and blue color indicates odd number chromosomes Full size image Genetic correlations between cancer and other traits Significant genetic correlations ( p < 0.05/228 = 0.0002) between the six cancers and 38 non-cancer traits reflected several known associations (Fig. 3 and Supplementary Data 3 ). We observed a strong genetic correlation between smoking and lung cancer ( r g = 0.56, se = 0.06), and similarly for head/neck cancer ( r g = 0.47, se = 0.08), both cancers having smoking as its primary risk factor [19] , [20] . Educational attainment was negatively genetically correlated with colorectal ( r g = −0.17, se = 0.04), head/neck ( r g = −0.42, se = 0.07), and lung cancer ( r g = −0.39, se=0.04) (all p < 5 × 10 −6 ). Body mass index (BMI) showed a positive genetic correlation with colorectal cancer ( r g = 0.15, se = 0.03) and also suggestive but weak negative correlations with prostate ( r g = −0.07, se = 0.03) and breast cancer ( r g = −0.06, se = 0.03). Lung cancer showed a negative genetic correlation with lung function ( r g = −0.15, se = 0.04) and age at natural menopause ( r g = −0.25, se = 0.05), and moderate positive genetic correlations with depressive symptoms ( r g = 0.25, se=0.06) and waist-to-hip ratio ( r g = 0.16, se = 0.04). Breast cancer showed a positive genetic correlation with schizophrenia ( r g = 0.14, se = 0.03). Fig. 3 Cross-trait genetic correlation ( r g ) analysis between cancers and non-cancer traits. The traits were divided into four categories: a Common phenotypes, b Metabolic or cardiovascular related traits, c Psychiatric traits, d Autoimmune inflammatory diseases. Pair-wise genetic correlations withstood Bonferroni corrections (228 tests) are marked with double asterisk (**), with estimates of correlation shown in the cells. Pair-wise genetic correlations with significance at p < 0.01 are marked with a single asterisk (*). The color of cells represents the magnitude of correlation Full size image We did not find evidence of genetic correlations between cancer and several previously suggested risk factors [21] , [22] , [23] including cardiovascular traits (coronary artery disease, hypertension, and blood pressure) or sleep characteristics (chronotype, duration, and insomnia). Further, we did not observe genetic correlations between cancer and circulating lipids (HDL, LDL, and triglycerides) or type 2 diabetes-related traits except a significant negative correlation between HDL and lung cancer ( r g = −0.14, se = 0.04). We observed no significant genetic correlation between breast cancer and age at menarche ( r g = −0.03, se = 0.03) or age at natural menopause ( r g = −0.01, se = 0.03). We also did not observe notable genetic correlations between cancer and autoimmune inflammatory diseases or height. Subtype analysis revealed that smoking and educational attainment showed genetic correlations with all lung cancer subtypes (Supplementary Data 3 ). Educational attainment, forced vital capacity and depressive symptoms showed genetic correlations with ER− but not ER + breast cancer, whilst the observed genetic correlation between schizophrenia and breast cancer was limited to ER + disease, and the genetic correlation between depressive symptoms and lung cancer was observed only for lung squamous cell carcinoma. We further assessed the support for mediated or pleiotropic causal models for non-cancer traits and cancer using the correlation between trait-specific effect sizes of genome-wide significant SNPs for pairs of phenotypes. We detected four putative directional genetic correlations (defined as p < 0.05 from a likelihood ratio (LR) comparing the best non-causal model to the best causal model) (Fig. 4 ), where SNPs associated with the non-cancer trait showed correlated effect estimates with cancer but the reverse was not true (circulating HDL concentrations and breast cancer, LR non-causal vs. causal = 0.04, schizophrenia and breast cancer, LR non-causal vs. causal = 0.003, age at natural menopause and breast cancer, LR non-causal vs. causal = 0.04, and lupus and prostate cancer, LR non-causal vs. causal = 0.0006). Fig. 4 Putative directional relationships between cancers and traits. For each cancer–trait pair identified as candidates to be related in a causal manner, the plots show trait-specific effect sizes (beta coefficients) of the included genetic variants. Gray lines represent the relevant standard errors. a HDL and breast cancer. Trait-specific effect sizes for HDL and breast cancer are shown for SNPs associated with HDL levels (left) and breast cancer (right). b Schizophrenia and breast cancer. Trait-specific effect sizes for schizophrenia and breast cancer are shown for SNPs associated with schizophrenia (left) and breast cancer (right). c Age at natural menopause and breast cancer. Trait-specific effect sizes for age at natural menopause and breast cancer are shown for SNPs associated with age at natural menopause (left) and breast cancer (right). d Lupus and prostate cancer. Trait-specific effect sizes for lupus and prostate cancer are shown for SNPs associated with lupus (left) and prostate cancer (right) Full size image Functional enrichment analysis of cancer heritability Finally, we partitioned SNP-heritability of each cancer by using 24 genomic functional annotations (the baseline-LD model described in Gazal et al. [24] ) and 220 cell-type-specific histone mark annotations (the cell-type-specific model described in Finucane et al. [14] ). Meta-analysis across the six cancers revealed statistically significant enrichments for multiple functional categories. 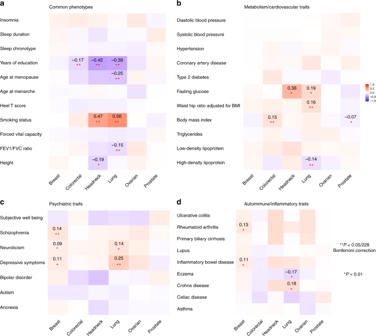Fig. 3 Cross-trait genetic correlation (rg) analysis between cancers and non-cancer traits. The traits were divided into four categories:aCommon phenotypes,bMetabolic or cardiovascular related traits,cPsychiatric traits,dAutoimmune inflammatory diseases. Pair-wise genetic correlations withstood Bonferroni corrections (228 tests) are marked with double asterisk (**), with estimates of correlation shown in the cells. Pair-wise genetic correlations with significance atp< 0.01 are marked with a single asterisk (*). The color of cells represents the magnitude of correlation We observed the highest enrichment for conserved regions (Table 1 , Supplementary Table 3 ) which overlapped with only 2.6% of SNPs but explained 25% of cancer SNP-heritability (9.8-fold enrichment, p = 2.3 × 10 −5 ). Transcription factor binding sites showed the second highest enrichment (4.0-fold, 13% of SNPs explaining 40% of SNP-heritability, p = 1.4 × 10 −7 ). Further, super-enhancers (groups of putative enhancers in close genomic proximity with unusually high levels of mediator binding) showed a significant 2.6-fold enrichment ( p = 2.0 × 10 −20 ). Additional enhancers, including regular enhancers (3.2-fold), weak enhancers (3.1-fold) and FANTOM5 enhancers (3.1-fold), presented similar enrichments but were not statistically significant. In addition, multiple histone modifications of epigenetic markers H3K9ac, H3K4me3, and H3K27ac, were all significantly enriched for cancer heritability. Repressed regions exhibited depletion (0.34-fold, p = 1.2 × 10 −6 ). Enrichment analysis of functional categories for each cancer and cancer subtype are shown in Fig. 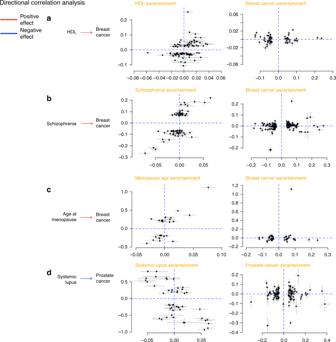Fig. 4 Putative directional relationships between cancers and traits. For each cancer–trait pair identified as candidates to be related in a causal manner, the plots show trait-specific effect sizes (beta coefficients) of the included genetic variants. Gray lines represent the relevant standard errors.aHDL and breast cancer. Trait-specific effect sizes for HDL and breast cancer are shown for SNPs associated with HDL levels (left) and breast cancer (right).bSchizophrenia and breast cancer. Trait-specific effect sizes for schizophrenia and breast cancer are shown for SNPs associated with schizophrenia (left) and breast cancer (right).cAge at natural menopause and breast cancer. Trait-specific effect sizes for age at natural menopause and breast cancer are shown for SNPs associated with age at natural menopause (left) and breast cancer (right).dLupus and prostate cancer. Trait-specific effect sizes for lupus and prostate cancer are shown for SNPs associated with lupus (left) and prostate cancer (right) 5 and Supplementary Table 4 . Table 1 Significant enrichment estimates of genomic functional categories, meta-analyzed across six cancer sites Full size table Fig. 5 Enrichment p -values of 24 non-cell-type-specific functional categories over six cancer types. The x -axis represents each of the 24 functional categories, y -axis represents log-transformed p -values of enrichment. Annotations with statistical significance after Bonferroni corrections ( p < 0.05/24) were plotted in orange, otherwise blue. The horizontal gray dash line indicates p -threshold of 0.05; horizontal red dash line indicates p -threshold of 0.05/24. From top to bottom are six panels representing six cancers: breast cancer, colorectal cancer, head/neck cancer, lung cancer, ovarian cancer, and prostate cancer. TSS transcription start site, UTR untranslated region, TFBS transcription factor binding sites, DHS DNase I hypersensitive sites, DGF digital genomic foot printing, CTCF CCCTC-binding factor Full size image Overall, cell-type-specific analysis of histone marks identified significant enrichments specific to individual cancers (Supplementary Fig. 2 ). For breast cancer, 3 out of 8 statistically significant tissues were adipose nuclei (H3K4me1, H3K9ac) and breast myoepithelial (H3K4me1) cells. For colorectal cancer, 15 out of the 18 statistically significant enrichments were observed in either colon or rectal tissues (colon/rectal mucosa, duodenum mucosa, small/large intestine, and colon smooth muscle). We observed no significant enrichments for head/neck, lung, and ovarian cancer, but we noted that for both lung (9 out of 10) and ovarian cancer (6 out of 10), the most enriched cell types were immune cells; while in head/neck cancer, 6 out of 10 most highly enriched cell types belonged to CNS (Supplementary Fig. 3 , Supplementary Data 4 ). Cell-type-specific analysis for cancer subtypes are shown in Supplementary Data 5 . Comparing cell-type-specific enrichment for cancers to the additional 38 non-cancer traits revealed notably differential clustering patterns (Supplementary Fig. 4 ). Breast, colorectal, and prostate cancer showed enrichment mostly for adipose and epithelial tissues, in contrast to autoimmune diseases (enriched for immune/hematopoietic cells) or psychiatric disorders (enriched for brain tissues). We performed a comprehensive analysis quantifying the heritability and genetic correlation of six cancers, leveraging summary statistics from the largest cancer GWAS conducted to date. Our study demonstrates shared genetic components across multiple cancer types. These results contrast with a prior study conducted by Sampson et al. which reported an overall negligible genetic correlation among common solid tumors [9] . Our results are, however, in line with a recent study, [16] which analyzed a subset of the data included here, and identified a significant genetic correlation between lung and colorectal cancer. Our data support, and for the first time quantify, the strong genetic correlation ( r g = 0.57) between lung and head/neck cancer, two cancers linked to tobacco use [20] , [25] . We also for the first time observed a significant genetic correlation between breast and ovarian cancer ( r g = 0.24), two cancers that are known to share rare genetic factors including BRCA1 / 2 mutations, and environmental exposures associated with endogenous and exogenous hormone exposures [26] . Prostate cancer is also considered as hormone-dependent and associated with BRCA1/2 mutations, but interestingly, we only observed a nominally significant and modest ( r g = 0.07) genetic correlation between breast and prostate cancer, while ovarian and prostate cancer showed no genetic correlation ( r g = 0.02, se = 0.07). Our large sample sizes allowed us to conduct well-powered analyses for cancer subtypes. While head/neck cancer showed negligible genetic correlation with overall ( r g = 0.03, se = 0.06) and ER + breast cancer ( r g = −0.02, se = 0.07), it showed a stronger genetic correlation with ER− breast cancer ( r g = 0.21, se = 0.09). Similarly, lung cancer showed a statistically more pronounced genetic correlation with ER− ( r g = 0.29, se = 0.06) than ER + breast cancer ( r g = 0.13, se = 0.04). A recent pooled analysis of smoking and breast cancer risk demonstrated a smoking-related increased risk for ER + but not for ER− breast cancer [27] , and thus it is unlikely that the stronger genetic correlation between ER− subtype and lung and head/neck cancer is due to smoking behavior. Perhaps surprisingly, despite literature suggesting substantial similarities between ER− breast cancer and serous ovarian cancer in particular [28] , we did not observe statistically significant different genetic correlations between ER− or ER + breast cancer and serous ovarian cancer ( r g = 0.17, se = 0.08 vs. r g = 0.11, se = 0.06). This suggests that rare high penetrance variants may play a more important role in driving the similarities behind ER− breast cancer and serous ovarian cancer than common genetic variation. Heritability analysis confirms that common cancers have a polygenic component that involves a large number of variants. Although susceptibility variants identified at genome-wide significance explain an appreciable fraction of the heritability for some cancers, we estimate that the majority of the polygenic effect is attributable to other, yet undiscovered variants, presumably with effects that are too weak to have been identified with current sample sizes. We found the genetic component that could be attributed to genome-wide significant loci varied greatly from ~0% for head/neck cancer to ~50% for breast and prostate cancer. These results reflect in part the strong correlation between number of GWAS-identified loci and sample size, as we had more than twice as many breast and prostate cancer samples compared to the other cancers. One corollary is that larger GWAS are likely to identify new susceptibility loci that could help our understanding of disease development, improve prediction power of genetic risk scores and hence contribute to screening and personalized risk prediction [29] . Among the genetic correlations between cancer and non-cancer traits, we observed positive correlations for psychiatric disorders (depressive symptoms, schizophrenia) with lung and breast cancer, where findings from epidemiological studies have been suggestive but inconclusive. It has been proposed that the linkage between psychiatric traits and cancers are more likely to be mediated through cancer-associated risk phenotypes such as smoking, excessive alcohol consumption in depressed populations [30] , and reduced fertility patterns (e.g., nulliparous) in psychiatric populations [31] . Detailed analyses considering confounding traits like reproductive history and smoking are needed to make inference about the mechanisms involved. GWAS have identified pleiotropic regions influencing both lung cancer and nicotine dependence, such as 15q25.1 [32] , [33] . In line with those results, we identified a strong genetic correlation between smoking and both lung ( r g = 0.56) and head/neck cancer ( r g = 0.47). It remains unclear whether this genetic correlation is completely explained by the direct influence of smoking or if the shared genetic component affects the traits through separate pathways. Interestingly, a genetic correlation ( r g = 0.35, se = 0.14) between lung and bladder cancer, another smoking-associated cancer, has been identified previously [9] . Due to the small numbers of GWAS-identified smoking-associated SNPs, we were unable to assess a directional correlation between smoking and cancer, but we expect such analyses to become feasible as additional smoking-related SNPs are identified. We found modest positive, yet significant genetic correlations between adiposity-related measures (as reflected by waist-to-hip ratio, circulating HDL levels and BMI) and both colorectal and lung cancer, but negative genetic correlations between BMI and prostate and breast cancer, consistent with previous reported findings [34] and reinforce the complex dynamics between obesity and cancer where multiple factors including age, smoking, endogenous hormones and reproductive status play a role. We did not observe genetic correlations between breast cancer and age at menarche or age at natural menopause. These null observations were largely driven by ER + breast cancer (ER + : r g = 0.006, se = 0.03 vs. ER−: r g = −0.09, se = 0.04 for age at menarche. ER + : r g = 0.0005, se = 0.04 vs. ER−: r g = −0.10, se = 0.05 for age at natural menopause), and were unexpected given that both factors play pivotal roles in breast cancer etiology [35] and previous Mendelian randomization (MR) analyses have identified a link [36] , [37] . An important difference between genetic correlation and MR analyses is that the latter only considers genome-wide significant SNPs while the former incorporates the entire genome. It is possible that a relatively small overlap in strongly associated SNPs can result in significant MR results despite low evidence of an overall genetic correlation. Indeed, the directional genetic correlations we observed for age at natural menopause, schizophrenia, and HDL with breast cancer, and for lupus with prostate cancer, highlight again that although an overall genetic correlation may be negligible, there can still be genetic links between traits. It is important to note that we cannot rule out unmeasured confounding, including the possibility that these genetic variants affect an intermediate phenotype that is pleiotropic for both target traits. Given the observational nature of our data, these putative causal directions should be interpreted with caution. Pan-cancer tumor-based studies have demonstrated that different cancers are sometimes driven by similar somatic functional events such as specific copy number abnormalities and mutations [38] , [39] . Our enrichment results of germline genetic across functional annotation data shed new light on the biological mechanisms leading to cancer development. The more pronounced enrichment identified for conserved regions compared with coding regions provides evidence for the biological importance of the former, which has been shown to be true for multiple traits [14] , [40] . Even though the biochemical function of many conserved regions remains uncharacterized, transcribed ultra-conserved regions have been found to be frequently located at fragile sites. Compared to normal cells, cancer cells have a unique spectrum of transcribed ultra-conservative regions, suggesting that variation in expression of these regions are involved in the malignant process [41] , [42] . These results bridge the link between germline and somatic genetics in cancer development, which was also observed in a recent breast cancer GWAS that has demonstrated a strong overlap between target genes for GWAS hits and somatic driver genes in breast tumors [43] . We also found a four-fold enrichment for transcription factor binding sites and a three-fold enrichment for super-enhancers, consistent with prior observations that breast cancer GWAS loci fall in enhancer regions involved in distal regulation of target genes [43] . Cell-type-specific analysis of histone marks demonstrated the importance of tissue specificity, primarily for colorectal and breast cancer. Further, our results suggest that immune cells are important for ovarian and lung cancer whilst CNS is important to head/neck cancer. Unfortunately, we did not have data on prostate-specific tissues, but we note that tissue-specific enrichment of prostate cancer heritability for epigenetic markers has been observed previously [10] . We note that generation of rich functional annotation is ongoing and we expect to include additional tissue-specific functional elements in our future work. Our study has several strengths. We were able to robustly quantify pair-wise genetic correlations between multiple cancers using the largest available cancer GWAS, comprising almost 600,000 samples across six major cancers and subtypes. We were also able to systematically assess the genetic correlations between cancer and 38 non-cancer traits. Notwithstanding the large sample sizes, several limitations need to be acknowledged. We did not have the sample sizes required to assess relevant cancer subgroups including oropharyngeal cancer, clear cell, mucinous and endometrioid ovarian cancer, or lung cancer among never smokers (each with ~2000 cases). In addition, we did not have access to GWAS summary statistics for pre- vs. post-menopausal breast cancer. We were not able to consider all cancer risk factors when selecting non-cancer traits, since some of the well-established risk factors such as infection were either not available, showed no evidence of heritability or were not based on adequate sample sizes for robust analyses. SNP-heritability varies with minor allele frequency, linkage disequilibrium, and genotype certainty; we note that approaches to estimate heritability leveraging GWAS data are constantly evolving. We also note that estimate variability needs to be taken into account when comparing the SNP-heritability with the classical twin-heritability, in particular for cancers with small sample sizes such as head/neck cancer (SNP-heritability varied between 5–14% and twin-heritability varied between 0–60%, although both point estimates were 9%). Further, our data were based on GWAS meta-analysis from multiple individual GWAS across European ancestry populations from Europe, Australia and the US. Intra-European ancestry differences are likely to be a source of bias. However, since we limited our analysis to SNPs with MAF > 1% and HapMap3 SNPs (which have proven to be well imputed across European ancestry populations), we believe that any population structure across cancers will have minimal effect on our results. Finally, as more non-European and multi-ethnic GWAS data become available, it is important to examine trans-ethnic genetic correlation in cancer. In conclusion, results from our comprehensive analysis of heritability and genetic correlations across six cancer types indicate that solid tumors arising from different tissues share common germline genetic influences. Our results also demonstrate evidence for common genetic risk sharing between cancers and smoking, psychiatric, and metabolic traits. In addition, functional components of the genome, particularly conserved and regulatory regions, are significant contributors to cancer heritability across multiple cancer types. Our results provide a basis and direction for future cross-cancer studies aiming to further explore the biological mechanisms underlying cancer development. Studies and quality control We used summary statistics from six cancer GWASs based on a total of 597,534 participants of European ancestry. Cancer-specific sample sizes were: breast cancer: 122,977 cases/105,974 controls; colorectal cancer: 36,948/30,864; head/neck cancer (oral and oropharyngeal cancers): 5452/5984; lung cancer: 29,266/56,450; ovarian cancer: 22,406/40,941; prostate cancer: 79,166/61,106. These data were generated through the joint efforts of multiple consortia. Details on study characteristics and subjects contributed to each cancer-specific GWAS summary dataset have been described elsewhere [43] , [44] , [45] , [46] , [47] , [48] , [49] . SNPs were imputed to the 1000 Genomes Project reference panel (1KGP) using a standardized protocol for all cancer types [18] . We included autosomal SNPs with a minor allele frequency (MAF) larger than 1% and present in HapMap3 (N SNPs = ~1 million) because those SNPs are usually well imputed in most studies (note that excluding sex chromosomes could reduce the overall heritability estimates). 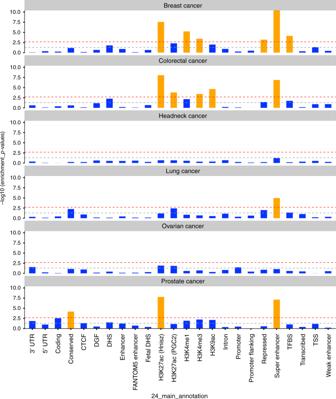Fig. 5 Enrichmentp-values of 24 non-cell-type-specific functional categories over six cancer types. Thex-axis represents each of the 24 functional categories,y-axis represents log-transformedp-values of enrichment. Annotations with statistical significance after Bonferroni corrections (p< 0.05/24) were plotted in orange, otherwise blue. The horizontal gray dash line indicatesp-threshold of 0.05; horizontal red dash line indicatesp-threshold of 0.05/24. From top to bottom are six panels representing six cancers: breast cancer, colorectal cancer, head/neck cancer, lung cancer, ovarian cancer, and prostate cancer. TSS transcription start site, UTR untranslated region, TFBS transcription factor binding sites, DHS DNase I hypersensitive sites, DGF digital genomic foot printing, CTCF CCCTC-binding factor A brief overview of the quality control in each cancer dataset are presented in Supplementary Table 5 . For some of the cancers, we further obtained summary statistics data on subtypes (ER + and ER− breast cancer; lung adenocarcinoma, and squamous cell carcinoma; serous invasive ovarian cancer and advanced stage prostate cancer, defined as metastatic disease or Gleason score ≥ 8 or PSA > 100 or prostate cancer death). Sample sizes and more details shown in Supplementary Table 1 . We additionally assembled European ancestry GWAS summary statistics from 38 traits, which spanned a wide range of phenotypes including anthropometric (e.g., height and body mass index (BMI)), psychiatric disorder (e.g., depressive symptoms and schizophrenia), and autoimmune disease (e.g., rheumatoid arthritis and celiac disease) (Supplementary Table 6 ). We calculated trait-specific SNP-heritability and restricted our analysis to traits with a heritable component (Supplementary Table 7 ) [14] . We removed the major histocompatibility complex (MHC) region from all analysis because of its unusual LD and genetic architecture. Estimation of SNP-heritability and genetic correlation We estimated the SNP-heritability due to genotyped and imputed SNPs ( \(h_g^2\) , the proportion of phenotypic variance causally explained by common SNPs) of each cancer using LDSC [15] . Briefly, this method is based on the relationship between LD score and χ 2 -statistics: 
    E[ χ _j^2] ≈N_jh_g^2/Ml_j + 1
 (1) where \(E\left[ {\chi _j^2} \right]\) denotes the expected χ 2 -statistics for the association between the outcome and SNP j , N j is the study sample size available for SNP j , M is the total numbers of variants and l j denotes the LD score of SNP j defined as \(l_j = \mathop {\sum }\limits_k r^2\left( {j,k} \right)\) ( k denotes other variants within the LD region). Note that the quantity estimated by LDSC is the causal heritability of common SNPs, which is different from the SNP-heritability as defined in Yang et al. [17] . To estimate \(h_g^2\) attributable to undiscovered loci, we identified SNPs that were associated with a given cancer at genome-wide significance ( p < 5 × 10 −8 ) and removed all SNPs within (+/−) 500,000 base-pairs of those loci prior to calculation (number of regions (+/− 500 kb) for each cancer that reach the 5 × 10 −8 threshold and measures of effect size are shown in Supplementary Data 1 ). We also converted the SNP-heritability from observed scale to liability scale by incorporating sample prevalence ( P ) and population prevalence ( F ) of each cancer: 
    h_liability^2 = h_observed^2F( 1 - F)/ϕ( Φ^ - 1( F ))^2F( 1 - F)/P( 1 - P)
 (2) We subsequently calculated the genome-wide genetic correlations ( r g ) between different cancers, and between cancers and non-cancer traits, using an algorithm [14] : 
    E[ β _jγ _j] = √(N_1N_2) r_g/Ml_j + N_sr/√(N_1N_2)
 (3) where β j and γ j are the effect sizes of SNP j on traits 1 and 2, r g is the genetic covariance, M is number of SNPs, N 1 and N 2 are the sample sizes for trait 1 and 2, N s is the number of overlapping samples, r is the phenotypic correlation in overlapping samples and l j is the LD score defined as above. For genetic correlation between 6 cancers, the significance level is 0.05/15 = 0.003; for genetic correlation between 6 cancers and 38 traits, the significance level is 0.05/(6 × 38) = 0.0002. Overall genetic correlations as estimated by LDSC are based on aggregated information across all variants in the genome. It is possible that even though two traits show negligible overall genetic correlation, there are specific regions in the genome that contribute to both traits. We therefore examined local genetic correlations between cancer pairs using ρ-HESS [50] , an algorithm which partitions the whole genome into 1703 regions based on LD-pattern of European populations and quantifies correlation between pairs of traits due to genetic variation restricted to these genomic regions. Local genetic correlation was considered statistically significant if p < 0.05/1,703 = 2.9 × 10 −5 . In particular, we assessed the local genetic correlations for previously reported pleiotropic regions [18] , [51] known to harbor SNPs affecting multiple cancers. Directional genetic correlation analysis In addition to the genetic correlation analysis, which reflects overall genetic overlaps, we also attempted to identify directions of potential genetic correlations using a subset of SNPs as proposed by Pickrell et al. [52] . The method adopts the following assumption: if a trait X influences trait Y, then SNPs influencing X should also influence Y, and the SNP-specific effect sizes for the two traits should be correlated. Further, since Y does not influence X, but could be influenced by mechanisms independent of X, genetic variants that influence Y do not necessarily influence X. Based on this assumption, the method proposes two causal models and two non-causal models; and calculates the relative likelihood ratio (LR) of the best non-causal model compared to the best causal model. We determined significant SNPs for each given cancer or trait in two independent ways, (1) LD pruned SNPs: we selected genome-wide significant ( p < 5 × 10 −8 ) SNPs and pruned on LD-pattern in the European populations in Phase1 of 1KGP; (2) posterior probability of association (PPA) SNPs: we used a method implemented in fgwas [53] , which splits the genome into independent blocks based on LD patterns in 1KGP and estimates the prior probability that any block contains an association. The model outputs posterior probability that the region contains a variant that influences the trait. We selected the lead SNP from each of the regions with a PPA of at least 0.9. We scanned through all pairs of cancers and traits to identify directional correlations. Only pairs of traits with evidence of directional correlations (LR comparing the best non-causal model over the best causal model < 0.05) and without evidence of heteroscedasticity (pleiotropic effects) [54] were reported as relatively more likely to exhibit mediated causation. Functional partitioning of SNP-heritability To assess the importance of specific functional annotations in SNP-heritability across cancers, we partitioned the cancer-specific heritability using stratified-LDSC [14] . This method partitions SNPs into functional categories and calculates category-specific enrichments based on the assumption that a category of SNPs is enriched for heritability if SNPs with high LD to that category have higher χ 2 statistics than SNPs with low LD to that category. The analysis was performed using two models [14] , [24] . 1. A full baseline-LD model including 24 publicly available annotations that are not specific to any cell type. When performing this model, we adjusted for MAF via MAF-stratified quantile-normalized LD score, and other LD-related annotations such as predicted allele age and recombination rate, as implemented by Gazal et al. [24] . Briefly, the 24 annotations included coding, 3′UTR and 5′UTR, promoter and intronic regions, obtained from UCSC Genome Browser and post-processed by Gusev et al. [55] ; the histone marks mono-methylation (H3K4me1) and tri-methylation of histone H3 at lysine 4 (H3K4me3), acetylation of histone H3 at lysine 9 (H3K9ac) processed by Trynka et al. [56] , [57] , [58] and two versions of acetylation of histone H3 at lysine 27 (H3K27ac, one version processed by Hnisz et al. [59] , another used by the Psychiatric Genomics Consortium (PGC) [60] ); open chromatin, as reflected by DNase I hypersensitivity sites (DHSs and fetal DHSs) [55] , obtained as a combination of ENCODE and Roadmap Epigenomics data, processed by Trynka et al. [58] ; combined chromHMM and Segway predictions obtained from Hoffman et al. [61] , which make use of many annotations to produce a single partition of the genome into seven underlying chromatin states (The CCCTC-binding factor (CTCF), promoter-flanking, transcribed, transcription start site (TSS), strong enhancer, weak enhancer categories, and the repressed category); regions that are conserved in mammals, obtained from Lindblad-Toh et al. [40] and post-processed by Ward and Kellis [62] ; super-enhancers, which are large clusters of highly active enhancers, obtained from Hnisz et al. [59] ; FANTOM5 enhancers with balanced bi-directional capped transcripts identified using cap analysis of gene expression in the FANTOM5 panel of samples, obtained from Andersson et al. [63] ; digital genomic footprint (DGF) and transcription factor binding site (TFBS) annotations obtained from ENCODE and post-processed by Gusev et al. [55] 2. In addition to the baseline-LD model, we also performed analyses using 220 cell-type-specific annotations for the four histone marks H3K4me1, H3K4me3, H3K9ac, and H3K27ac. Each cell-type-specific annotation corresponds to a histone mark in a single cell type (for example, H3K27ac in CD19 immune cells), and there were 220 such annotations in total. We further divided these 220 cell-type-specific annotations into 10 groups (adrenal and pancreas, central nervous system (CNS), cardiovascular, connective and bone, gastrointestinal, immune and hematopoietic, kidney, liver, skeletal muscle, and other) by taking a union of the cell-type-specific annotations within each group (for example, SNPs with any of the four histone modifications in any hematopoietic and immune cells were considered as one big category). When generating the cell-type-specific models, we added annotations individually to the baseline model, creating 220 separate models. We performed a random-effects meta-analysis of the proportion of heritability over six cancers for each functional category. We set significance thresholds for individual annotations at p < 0.05/24 for baseline model and at p < 0.05/220 for cell-type-specific annotation.